The genomics of selection in dogs and the parallel evolution between dogs and humans The genetic bases of demographic changes and artificial selection underlying domestication are of great interest in evolutionary biology. Here we perform whole-genome sequencing of multiple grey wolves, Chinese indigenous dogs and dogs of diverse breeds. Demographic analysis show that the split between wolves and Chinese indigenous dogs occurred 32,000 years ago and that the subsequent bottlenecks were mild. Therefore, dogs may have been under human selection over a much longer time than previously concluded, based on molecular data, perhaps by initially scavenging with humans. Population genetic analysis identifies a list of genes under positive selection during domestication, which overlaps extensively with the corresponding list of positively selected genes in humans. Parallel evolution is most apparent in genes for digestion and metabolism, neurological process and cancer. Our study, for the first time, draws together humans and dogs in their recent genomic evolution. The genetic basis of animal and plant domestication is an interesting question that is also of practical value [1] . The remarkable diversity in the physical and behavioural traits in dogs is one of the most interesting examples of domestication [2] , [3] , [4] , [5] . The evolution of dogs is often depicted as a two-stage process. In the first stage, dogs were domesticated from their wild relatives, possibly the grey wolves of Southeast Asia [6] , [7] , [8] , [9] , [10] , [11] . Ever since then, dogs and humans lived commensally sharing the same living environments and food resources [3] . In the second stage spanning the last few hundred years, intensive breeding programs have created many modern breeds and selected for an assortment of human favourable characters [12] . Many studies have focused on the genetic basis of phenotypic variation in modern breeds [13] , [14] . In contrast, the genetic changes associated with the transition from wolves to ancestral dogs have received far less attention. Previous studies using mtDNA and Y chromosome data found that the indigenous dogs from China, together with several dog breeds that originated from Southeast Asia/China (often designated as ancient breeds), have the highest genetic diversity and are the basal lineages connecting to the wild grey wolves [6] , [9] , [10] . Whole-genome analysis using single-nucleotide polymorphism (SNP) chips among a large number of canids also revealed a closer relationship between these ancient breeds and the wild wolves [4] , [5] . Thus, the native dogs of South China are likely the most primitive form of dogs and may represent the product of the first stage of domestication [6] , [9] , [10] . Coupled with the availability of the dog genome and the rapid advances in sequencing technology, the study of the native dog populations in China may shed considerable light on the early history of dog domestication. In this study, we perform whole-genome sequencing of four grey wolves, three Chinese indigenous dogs and three modern breeds, and identify 13.92 million SNPs and 3.02 million small indels. Genome-wide analysis shows a general trend of decreasing diversity from wolves to Chinese indigenous dogs to dog breeds. Demographic analysis reveals a population split between wolves and Chinese indigenous dogs that is as old as 32,000 years ago and that subsequent bottlenecks are rather mild, suggesting that dogs may have been domesticated initially through their scavenging with humans. Population genetic analysis identifies 311 genes under positive selection with strong enrichment in the sexual reproduction, digestion and metabolism, and neurological processes. Interestingly, this list of genes is found to overlap extensively with those that have been selected in humans. The overlap in sets is most apparent for genes involved in digestion and metabolism, neurological process and cancer. Our study, for the first time, reveals striking parallelism in the recent evolution of dogs and humans. Sample collection and sequencing Four grey wolves from locations across Eurasia and three Chinese indigenous dogs from Southwest China were collected for this work ( Fig. 1a ). 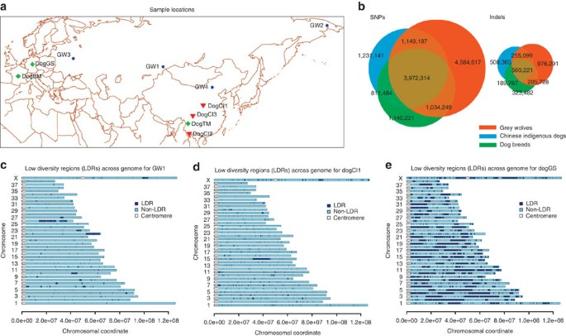Figure 1: Sampling and diversity information of the dog and wolf individuals. (a) The geographic locations for the four grey wolves (GW1–4), three Chinese indigenous dogs (dogCI1–3), two European dog breeds (dogGS: Germany Shepherd, and dogBM: Belgium Malinois), and one Tibetan Mastiff (dogTM) used in this study are indicated. (b) SNP and small indels overlapping between the three different populations, respectively, (wolves, Chinese indigenous dogs and dog breeds). (c) Low-diversity regions (LDRs) plotted across the genome for the grey wolf 1. The cutoff value for LDRs is 0.00005. (d) LDRs plotted across the genome for the Chinese indigenous dog 1. (e) LDRs plotted across the genome for the German shepherd. LDR plots for the other individuals are shown in theSupplementary Fig. S3. In addition, we also sequenced dogs from three breeds, one German Shepherd, one Belgium Malinois and one Tibetan Mastiff ( Table 1 ). Of the four grey wolves and six dogs we sequenced, the effective throughput for each individual ranges from 8.92X to 13.56X ( Supplementary Table S1 ). Sanger sequence data for the reference Boxer genome was also downloaded from the NCBI trace archive for subsequent analysis [7] . Figure 1: Sampling and diversity information of the dog and wolf individuals. ( a ) The geographic locations for the four grey wolves (GW1–4), three Chinese indigenous dogs (dogCI1–3), two European dog breeds (dogGS: Germany Shepherd, and dogBM: Belgium Malinois), and one Tibetan Mastiff (dogTM) used in this study are indicated. ( b ) SNP and small indels overlapping between the three different populations, respectively, (wolves, Chinese indigenous dogs and dog breeds). ( c ) Low-diversity regions (LDRs) plotted across the genome for the grey wolf 1. The cutoff value for LDRs is 0.00005. ( d ) LDRs plotted across the genome for the Chinese indigenous dog 1. ( e ) LDRs plotted across the genome for the German shepherd. LDR plots for the other individuals are shown in the Supplementary Fig. S3 . Full size image Table 1 Sample and sequencing throughput for all 11 individuals. Full size table After aligning the short reads to the reference genome, we identified single-nucleotide polymorphisms and small insertions and deletions (length <50) for all the individuals (Details of the data flow are presented in the Supplementary Fig. S1 ). Across the 11 individual genomes, a total of 13,923,223 SNPs were identified, of which 10,740,377 were found within the 4 wolves, 7,164,136 within the 3 Chinese indigenous dogs and 6,958,268 within the 4 breed dogs ( Fig. 1b ). A parallel analysis was also conducted for small indels, which yielded a similar pattern with the greatest number found in wolves and least within the breed dogs ( Fig. 1b ). Through experimental verification, we found current scheme in identifying variants maintains high levels of sensitivity with very limited amount of false positives. For example, we found that the overall false positive rate is less than 5% and for non-singleton polymorphism, genome-wide false negative is less than 10% ( Supplementary Note 1 ). Genetic diversity and population structure Using the heterozygous sites called within a diploid organism, we performed a sliding window analysis of the genetic diversity θ (4 Nμ) along the genome for each individual. Interestingly, the genetic diversity shows a decreasing order from wild wolves, to Chinese indigenous dogs and then modern breeds ( Table 1 ). This trend is most evident when we partition the genome into segments of very low diversity and plot this pattern across the genome ( Fig. 1c–e ). This decreasing order matches with the expectation from a two-stage history where Chinese indigenous dogs represent the groups following the first domestication event. Using the phased genotypes, linkage disequilibrium, in terms of the correlation coefficient ( r 2 ), was calculated for wolves and the Chinese indigenous dog populations. As seen in Fig. 2a , linkage disequilibrium decreases rapidly for both wolves and the Chinese indigenous dogs. Within distances as short as 5 kb, levels of correlation decrease very rapidly to below 0.2, with this trend being slightly stronger in the wolves than in the Chinese indigenous dogs. The similarity in linkage disequilibrium observed here suggests that a relative weak population bottleneck might have occurred during dog domestication. 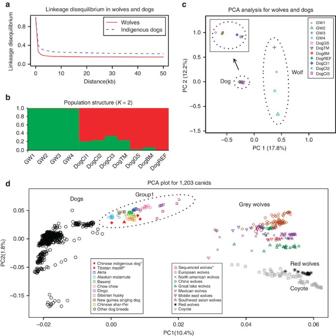Figure 2: Population structure and principle component analysis. (a) Correlation coefficients (r2) were calculated for the wolf/dog populations over 50 kb windows. (b) Structure analysis on all the individuals withK=2. (c) Principle component plots for the first two PCs for all 11 individuals. Inset figure is a zoomed-in version of the dog group. (d) Principle component plot for 1203 canids including our data and individuals from a previous study4. The group 1 is the cluster of dogs that are closest to grey wolves. Figure 2: Population structure and principle component analysis. ( a ) Correlation coefficients ( r 2 ) were calculated for the wolf/dog populations over 50 kb windows. ( b ) Structure analysis on all the individuals with K =2. ( c ) Principle component plots for the first two PCs for all 11 individuals. Inset figure is a zoomed-in version of the dog group. ( d ) Principle component plot for 1203 canids including our data and individuals from a previous study [4] . The group 1 is the cluster of dogs that are closest to grey wolves. Full size image Given the genotypes across the genomes, we did Bayesian clustering inferences by partitioning the individuals into K =2 and K =3 groups. As seen from Fig. 2b , when we try to cluster the individuals into two groups, the first cluster separates all of the grey wolves from the dogs. Interestingly, the Chinese indigenous dogs and the Tibetan Mastiff showed a closer relationship with the wolves. When we tried to partition the sample into three clusters, the analysis started to split the wolves into further groups, likely due to the higher distances within the wolves ( Supplementary Fig. S4 ). In order to further explore the relative relationships between these individuals, a principle component analysis with all the individuals were carried out. When plotting the first two principle components, dogs and wolves were separated as two distinct groups ( Fig. 2c ). Interestingly, all of the dogs clustered quite tightly together and distantly from the wolves, however, the Chinese dogs, including the Tibetan Mastiff, were located slightly closer to the wolves ( Fig. 2c inset). Previous studies, using SNP genotyping arrays, have surveyed the global distribution of genetic diversity across a large number of dogs and wolf-like canids. When we combined the sequenced individuals with the 1,191 canids surveyed previously [5] , we found that the Chinese native dogs, together with several dog breeds that originated from China/Southeast Asia, are among the first tier of individuals that is closest to the grey wolves ( Fig. 2d ). In addition, when we compared the Chinese indigenous groups with native dogs from other geographic regions (for example, African village dogs [15] ), Chinese indigenous dogs are also found to be much closer to wolves than native dogs from other places surveyed to date ( Supplementary Note 2 ). The close proximity of the Chinese indigenous dogs and breeds originated from Southeast Asia to grey wolves, together with the high genetic diversity observed in the Chinese native dogs, support a Southeast Asia origin for dogs [9] , [10] . Demographic history Using joint site frequency spectra generated after polarizing the polymorphisms with an outgroup species (a red wolf), we inferred the population demographic history under an isolation migration model [16] . As presented in Fig. 3 , the effective population size for the wolf was found to have been relatively stable. The inferred effective population size for the extant wolf population is very similar to that inferred for the ancestral population, with the extant population being 94% of the size of the ancestral population. Interestingly, during domestication, the Chinese indigenous dog population experienced a mild bottleneck and the effective population size was reduced to 16% of the ancestral population size. Following the bottleneck, the population size has been steadily increasing to about 32% of that of the ancestral wolf population, which is largely consistent with the mild reduction in genetic diversity and the slight increase in linkage disequilibrium observed in the Chinese native dogs relative to the wolves. 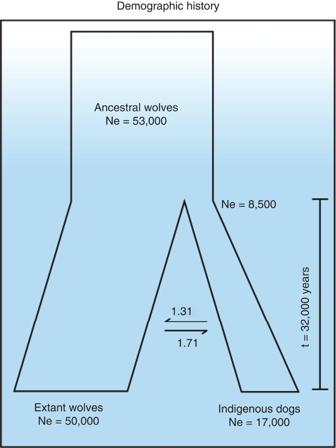Figure 3: Inferred demographic history for the wild wolves and the Chinese indigenous dogs. The extent and ancestral population sizes of two species are labelled. The migration rates between two populations are also labelled. As the current wolf’s average diversityθis equal to 0.00141 (θ=4 Neμ) per kb and current wolves have an effective size that is 94% of the ancestral population, we estimated that the effective population size of the ancestral wolf to be around 53,000. Figure 3: Inferred demographic history for the wild wolves and the Chinese indigenous dogs. The extent and ancestral population sizes of two species are labelled. The migration rates between two populations are also labelled. As the current wolf’s average diversity θ is equal to 0.00141 ( θ =4 N e μ) per kb and current wolves have an effective size that is 94% of the ancestral population, we estimated that the effective population size of the ancestral wolf to be around 53,000. Full size image With an assumed mutation rate of 2.2 × 10 −9 per year [17] and a generation time of 3 years, the effective population size of dogs at the beginning of the bottleneck is found to be around 8,500 and the effective size of the extant Chinese indigenous dog population to be around 17,000. Compared with other domesticated species, which typically experienced a population shrinkage of several magnitudes [18] , [19] , this level of population size reduction is rather weak. The population divergence time is estimated to be around 32,000 years ago, which is much older than previous estimates using mtDNA data [9] , [10] (see discussion). The estimated migration rate is not very large either. The migration rate from wolves to dogs (M dw ) is slightly higher than that estimated for the other direction. The estimated migration rate is compatible with our observation that dogs and wolves exist as two rather disjoint clusters in the PCA and structure analysis, and is also in agreement with previous observations that introgressive hybridization between dogs and wild wolves is rare [20] . Behavioural or selective constraints imposed on these two groups might be the limiting factor contributing to the low level of gene flow [20] , [21] . In order to access the statistical confidence in the estimated parameter values, we performed a non-parametric bootstrap test of the demographic history by resampling the SNPs to generate data sets of the same size with replacement. Under a variety of parameter settings, we found that the estimated values show a similar profile to that presented in Fig. 3 (see Methods as well as Supplementary Note 3 ), thus, the inferred demographic history shown here is supported with strong statistical confidence. Putatively selected genes during dog domestication As selection acting during the first stage of domestication should be shared among all dogs, we thus screened for candidate positively selected genes during dog domestication by looking for regions that show low diversity in all seven dogs and have high divergence between dogs and wolves. To avoid the possibility that a low-diversity segment was inherited from the wolf population, we filtered regions that showed relatively low diversity in wolves. Using a set of stringent conditions for positive selection, we identified the top 1% of the genome that is expected to be enriched for genes bearing the signature of positive selection. This portion of the genome is distributed across 198 segments carrying a total of 311 genes ( Supplementary Note 4 , Table S6 and Fig. S11 ). It is worth pointing out that demographic factors also tend to generate genetic patterns that mimic traces of positive selection [22] . Thus, this candidate list is expected to be enriched for genes responsible for the domestication of the dog. When genes were analysed by their broad classification in the Gene Ontology, three major categories, namely reproduction, digestion and metabolism and neurological process stood out strongly ( Table 2 ). Table 2 Gene ontology analysis of the candidate selected genes. Full size table Genes related to digestion and metabolism are particularly interesting. Multiple GO terms ranging from nutrient transport (for example, lipid) to the regulation of the digestion process (for example, cholesterol) are over-represented. An example of a gene that shows evidence of positive selection is the MGAM gene, an important maltase-glucoamylase in the final steps of starch digestion [23] . Along with the recent shared history between dogs and humans, in particular adopting an agricultural based living condition, large changes in the food source for dogs, during the transition from being a carnivore to an omnivore, might have been the driving force for the positive selection for these types of genes [24] . The other interesting GO category is the neurological process. Genes associated with nerve cells themselves (for example, axon) and their connectivity (for example, neuron projection) are among the set of genes that are positively selected. Strong selection on behaviour (for example, reducing aggression) and neurological traits (for example, complex interactions with human beings) is often involved in the first steps of animal domestication [25] . Genes of this class thus might underlie the processes that led to the successful domestication of the dog (see later sections). In addition, quite a few genes involved in sensing local environmental stimuli, for example, sound ( MYO3A ) and smell ( NCAM2 and OR2F1 ), are also on the list of selected genes. Large changes in the environment for dogs during domestication might have driven positive selection in these genes, some of which might reflect relaxed selective constraints on these proteins where loss of the activities of these genes is often adaptive (for example, less is more [26] ). Parallel selection in both human and dog Humans and dogs both experienced a suite of similar environments in the recent past. Natural selection, driven by convergent environmental pressures, might thus have worked on a similar set of genes in the two genomes. Genome-wide scans for positive selection in humans have been conducted using a wide variety of methods and data sets [27] , [28] . For example, Akey [22] compiled a collection of human genome regions that had been identified in at least two of nine different genome scans for positive selection [22] . To identify genes that may have been positively selected in parallel, we compared our list of positively selected genes in dogs with that from humans compiled in Akey [22] . Among the orthologous gene pairs between human and dog (a total of 17,661 gene pairs), 1,708 positively selected genes were identified for humans and 233 genes were found for dogs. Comparing these two data sets, 32 genes exist in the overlapping set between the two species (1.4 fold enrichment at a marginal significance of 0.03). Table 3 highlights genes of particular interests, with a full list summarized and presented in Supplementary Note 5 and Table S8 . Table 3 Positively selected genes found in both humans and dogs. Full size table A group of genes that appear to be under positive selection in both humans and dogs are those involved in digestion and metabolism. For example, two members of the ATP-binding cassette transporters superfamily, ABCG5 and ABCG8 , which have pivotal roles in the selective transport of dietary cholesterol [29] , were found on both lists. As domestication has lead to drastic changes in the proportions of plant food, relative to animal food, natural selection on these genes in both species is expected due to this shared evolutionary history. A second groups of genes selected in both species are those involved in neurological processes. An example of an interesting gene is SLC6A4 , an integral membrane protein that transports the neurotransmitter serotonin [30] and is a target of many psychomotor stimulants such as amphetamines and cocaine. Variation in this gene is responsible for a wide range of neurological pathogenic conditions such as aggressive behaviour [31] , obsessive-compulsive disorder [32] , depression and autism [33] , [34] . The most striking aspect is compulsive disorders, of which the two species share many similar phenotypes. Most interestingly, dogs respond similarly to the drugs that are used to treat humans (for example, clomipramine hydrochloride, a serotonin-reuptake inhibitor often also used as an anti-depressant drug), suggesting possible common genetic components for these behaviours in humans and dogs. Association studies have found that both the receptor and the downstream metabolite of SLC6A4 are correlated with aggressive behaviour in dogs [35] , [36] . The protein coded by SLC6A4 might underlie the genetic component of many neurological traits in both dogs and humans. Aside from genes involved in metabolism and neurological processes, the other most prevalent class of genes that overlap between the two species is the cancer related genes. A good example is MET , the mesenchymal epithelial transition factor, which is an important proto-oncogene. Abnormal activation of the MET pathway leads to a variety of tumours. Many other cancer related genes, including those involved in the cell cycle and apoptotic pathways, are present in our shared list, and are further discussed in Supplementary Note 5 . Chinese indigenous dogs might represent the missing link in dog domestication. The dense clustering of all dogs in the PCA plot, the closer distances between grey wolves and Chinese indigenous dogs together with the high genetic diversity within Chinese native dogs support a Southeast Asia origin for domesticated dogs. The whole-genome pattern also agrees with previous studies, based on mtDNA [9] , [10] and Y chromosome [6] data, as well as whole-genome SNP chip data [4] , [5] , that the Chinese indigenous dogs, and several ancient dog breeds originated from Southeastern Asia, are the basal groups connected to their wild ancestors. The Chinese indigenous dogs are likely one of the early groups that resulted from the first stage of dog domestication and were subsequently the source from which dog breeds were further selected. Thus, the study of the Chinese indigenous dog might hold great promise for illuminating the origin of dogs. The geographic location for dog domestication presented here, though quite strong, is not fully compatible with earlier studies that used wolves to identify the site of domestication. In particular, a previous study has argued for a Middle-Eastern origin of dogs based on the finding that Middle-Eastern wolves, as a group, seem to be closer to dogs than wolves from other places using the 48K SNP chip data [5] . However, the geographic distribution of wild wolves has been greatly affected by human activities in recent history. For example, the ancestral Chinese wolf, from which domesticated dogs may have originated, may already be extinct [9] . In addition, several wolves from Europe and Mexico are closer to dogs than the Middle-Eastern wolves ( Fig. 2d ), thus, it may be difficult to use patterns from extant wolves to infer domestication location. Nevertheless, it appears to be the case that the patterns revealed from wolves and dogs are not yet fully coherent. Further re-sequencing studies with more samples of wolves and indigenous dogs from around the world should bridge the two pictures drawn with dogs and wolves. The divergence time between the dog and wolf that we estimated implies a more ancient age for domestication than suggested by previous studies [9] , [10] . Even though the genetic evidence and fossil records in many parts of the world are still very preliminary [37] , archaeological remains of wolf-like canids, with some resemblance to the dog, as old as 30,000 years ago have recently been reported, although their status as dog is debated [38] , [39] , [40] , [41] . A deeper divergence and a mild population size reduction during domestication suggest an evolutionary trajectory for dogs that is often called self-domestication [42] . Early wolves might have been domesticated as scavengers that were attracted to live and hunt commensally with humans. With successive adaptive changes, these scavengers became progressively more prone to human custody. In light of this view, the domestication process might have been a continuous dynamic process, where dogs with extensive human contact were derived from these scavengers much latter when humans began to adopt an agricultural life style. Our study on positive selection in humans and dogs found an extraordinary amount of parallel evolution, which was likely driven by their similar environments. Natural selection acting on genes involved in neurological processes in both species is of particular interest. As domestication is often associated with large increases in population density and crowded living conditions, these ‘unfavourable’ environments might be the selective pressure that drove the rewiring of both species. Positive selection in neurological pathways, in particular the serotonin system, could be associated with the constant need for reduced aggression stemming from the crowded living environment [43] , [44] . Moreover, the complex intimate interactions between dogs and humans might have also driven some of the striking parallelism seen in these two species. Many genes that have undergone positive selection seem to be involved in similar diseases in both species. This could potentially be due to the pleiotropic effects of natural selection driven by the convergent environments (that is, antagonistic pleiotropy) [45] . Studying the genetic basis of these phenotypes among dog groups, in particular the disease associated traits including the many neurological diseases, might shed light on the genetic architecture of these disorders in humans. Parallel evolution happening in two species bestows on us an unprecedented opportunity to understand these traits by studying the evolution and the phenotypes in both species simultaneously. Interestingly, a companion study on hypoxic adaptation in Tibetan dogs also found strong evidence for parallel evolution between humans and dogs, implying that convergent evolution might be much more pervasive than observed here. Our best friend in the animal kingdom might provide us with one of the most enchanting systems for illuminating our understandings of human evolution and disease. Sample collection for whole-genome sequencing The genomes of four grey wolves and six domesticated dogs were sequenced for this study. The four grey wolves are from three different locations in Russia (Bryansk, Altai, and Chukotka), and one place in Inner Mongolia province of China. Of the six domesticated dogs sequenced, three are Chinese indigenous dogs. The Chinese indigenous dogs are the local dog populations that have lived in China for a long period of time and contain many ancestral polymorphisms retained since domestication from their wild ancestors [6] , [9] , [10] . The three indigenous dogs are sampled from the provinces of Shanxi, Yunnan and Sichuan. In addition to the three indigenous dogs, we also sequenced one individual each from three different modern dog breeds, the German shepherd, Belgian Malinois and Tibetan Mastiff. These breeds are selected from our sample collection and were chosen to broadly represent the breeds from Europe and Asia. The reference genomic sequence of a boxer was also extracted from the NCBI trace database for this study. Sample locations for the dogs and wolves are shown in Fig. 1a . Genome sequencing and mapping Total genomic DNA was extracted from blood samples using the phenol/chloroform method [9] . Whole-genome sequencing of each individual wolf and dog was performed on the Illumina GAIIx platform using a variety of fragment sizes ( Supplementary Table S1 ) and read lengths resulting in roughly 24.7–57.4 Gb of raw data for each individual. Details of the throughput and read lengths are summarized in Table 1 . Paired-end reads were aligned to the dog reference genome assembly CanFam2 [7] using the Burrows-Wheeler algorithm implemented in BWA-short [46] with default parameters. Trace data used for assembling the reference boxer genome was downloaded from NCBI and aligned to the reference genome with BWA-SW [47] . SNP calling and genotype estimation After sequence reads were mapped to the reference genome, mpileup files against the dog reference genome were generated using samtools [48] . After removing duplicated reads with same start/end points, candidate SNP positions were extracted based on the following conditions: (1) SNP quality greater than 20 and (2) no indel in the surrounding +/− 5 bp region [48] . After accumulating SNP positions, total coverage across all individuals was extracted. SNP positions with too low (total coverage <20) or two high coverage (total coverage >185) (possibly bad assembly or repetitive regions) were trimmed to ensure good quality in our final list. Given a SNP position, samtools was used to calculate the probability of each possible genotype conditioned on the observed reads from each individual. The genotype with maximal posterior probability was picked as the genotype for that locus. Identification of insertions and deletions The Pindel package [49] was used to curate a list of candidate indel positions together with the Dindel program. First, pair-end reads where one side could be uniquely mapped but not the other were collected. Unmapped reads were then spit and locally aligned according to library insert sizes. High quality candidate positions (single score s 1 >3 and probability score s 2 >30) were then extracted. Candidate positions in addition to information available in Dindel [50] were subsequently analysed where the local multiple sequence alignments were further refined and associated quality scores recomputed. High quality (filter: pass) candidates from the Dindel output were extracted as our final list of small insertions and deletions. Variant verification with the Sanger method Randomly selected genome segments covering a total of 382 SNPs from the nuclear genome were validated by traditional Sanger sequence technology in order to evaluate the sensitivity and specificity of the SNV calling strategy. PCR primers were designed based on the coordinates of the SNV locations. After a total of 614 amplifications, the PCR products were purified and sequenced by traditional Sanger sequence technology. Diversity estimation for each individual along the genome Watterson’s estimate of genetic diversity, which is based on the number of segregating sites were used to estimate the diversity across the genome [51] . For a single individual, the number of segregating sites is equivalent to the number of heterozygous sites in this individual within a segment of interest. The number of heterozygous sites was extracted for those candidate SNPs whose genotypes are most likely heterozygous. When the number of reads covering a genomic position is not very high, there is a possibility that one of the alleles was missed during sequencing. Watterson’s estimate of genetic diversity is modified to explicitly take into account this sampling effect [52] . Given the fact we have no less than 8X coverage of the genome, this correction was helpful, but not substantial. Phasing and linkage disequilibrium Given the genotype information across the genome for each individual, the program fastPHASE [53] was used to phase the genotypes into associated haplotypes with default parameters. Linkage disequilibrium was calculated using a custom written python script. We calculated the r 2 statistic, which is the correlation coefficient between two focal loci of interest. Population structure analysis SmartPCA program from the EIGENSOFT package (version 4.2) [54] was used to perform principle component analysis on the individuals that we sequenced. In addition, Structure (version 2.3.3) [55] was used to infer the population substructure among the samples. We varied the number for the population grouping parameter K to be 2 or 3 among different runs. SNP sets of different sizes after thinning the total number of SNPs with different distance conditions (that is, 100, 200 and 500 kb) between markers were implemented. The total length of the Markov Chain was set to be 1,100,000, of which 100,000 were burn-in steps. Population demographic history We inferred the population demographic history using methods implemented in the package ∂a∂i (version 1.60), which is based on the joint site frequency spectra between multiple populations [16] . Site frequency spectra is first extracted from our genotyping data and then polarized using a red wolf (an outgroup species) that we sequenced in a separate study. To avoid biases in the coding regions, only SNPs in the noncoding parts of the genome more than 5 kb from any coding region were extracted. Non-parametric bootstrapping was done by resampling (with replacement) the same number of SNPs from the total pool of SNPs. We assumed that the mutation rate per year is 2.2 × 10 −9 per year (ref. 17 ) and that the generation time is 3 years, thus the mutation rate per generation is 6.6 × 10 −9 per generation. Using the genetic diversity θ (4 N e μ) estimated across the genome and the mutation rate per generation, we can get a hold of the effective population size for the extant wolf population. Using the relative sizes of different populations ( Fig. 3 ) inferred from the demographic inference, we can calculate the population sizes of the other populations. The divergence time is calculated by combining the information from ∂a∂i and the population size estimates. In particular, the divergence time (τ) from ∂a∂i is measured in 2N e generations. The divergence time in years will be calculated as 2N e τ × 3. In the demographic analysis, we were setting the possible range of time of domestication to be between 0 and 0.3 (equivalence of 100,000 years, that is, before modern human’s migration out of Africa). In the bootstrap analysis, time spans of much larger range were also explored. In replicates where the estimated divergence time was far beyond the possible domestication time (that is, 250,000 years ago or further), those estimates were removed from the final results. This is equivalent to putting a hard bound on possible range of parameter estimates. Orthologous gene pair and enrichment analysis Gene orthologous relationship between human and dog was downloaded from Ensembl database ( www.ensembl.org ). In the enrichment analysis, the proportions of positively selected gene in two species were first computed (denoted as p 1 and p 2 ). The P- value was calculated as the proportion of simulated data sets that have equal or higher number of overlapped genes than the observed count. The simulation was done by randomly picking the same proportion of genes out of the total gene list, assuming independence among the two sets in human and dogs. Fst calculation and potential hitchhiking regions We used Weir and Cockerham [56] method to calculate Fst between wolf and dog populations using the inferred genotypes. After calculating the genome-wide diversity for each individual, the species specific mean diversities were calculated as the arithmetic mean across the seven individuals for the dog and the four individuals for wolves. Candidate hitchhiking regions were identified using three major criteria: (1) focal regions show reduced genetic diversity in the dog population (the bottom 5% quantile from the dog mean genome-wide distribution), (2) segments are not low-diversity regions in wolf (the bottom 20% quantile from the wolf mean genome-wide distribution), (3) there is a high divergence between the dog and wolf populations (we used top 95% quantile in the Fst distribution as the cutoff). Gene ontology Gene ontology enrichment test is performed using the Database for annotation, visualization and integrated discovery (DAVID) [57] . Associated transcript IDs were extracted from the Ensembl annotation. Accession codes: All short read data have been deposited into the Short Read Archive under the accession number SRA068869. How to cite this article: Wang, G.-d. et al . The genomics of selection in dogs and the parallel evolution between dogs and humans. Nat. Commun. 4:1860 doi: 10.1038/ncomms2814 (2013).